Ni-catalyzed hydroalkylation of olefins with N-sulfonyl amines Hydroalkylation, the direct addition of a C(sp 3 )–H bond across an olefin, is a desirable strategy to produce valuable, complex structural motifs in functional materials, pharmaceuticals, and natural products. Herein, we report a reliable method for accessing α-branched amines via nickel-catalyzed hydroalkylation reactions. Specifically, by using bis(cyclooctadiene)nickel (Ni(cod) 2 ) together with a phosphine ligand, we achieved a formal C(sp 3 )–H bond insertion reaction between olefins and N-sulfonyl amines without the need for an external hydride source. The amine not only provides the alkyl motif but also delivers hydride to the olefin by means of a nickel-engaged β–hydride elimination/reductive elimination process. This method provides a platform for constructing chiral α-branched amines by using a P-chiral ligand, demonstrating its potential utility in organic synthesis. Notably, a sulfonamidyl boronate complex formed in situ under basic conditions promotes ring-opening of the azanickellacycle reaction intermediate, leading to a significant improvement of the catalytic efficiency. Compounds featured with a carbon–carbon double bond serve as important precursors for complex aliphatic molecules because of their ready availability and versatility in transition-metal-catalyzed functionalizations [1] , [2] , [3] , [4] , [5] , [6] , [7] , [8] , [9] , [10] , [11] , [12] , [13] , [14] , [15] , [16] . In this respect, advances in nickel-complex-catalyzed hydrocarbonation of olefins have expanded the chemical space of accessible structures and enabled new synthetic disconnections [17] , [18] , [19] , [20] , [21] . Compared with hydroarylation [22] , [23] , [24] , [25] , [26] , [27] , [28] , [29] , [30] , [31] , [32] , [33] , [34] and hydroalkenylation [26] , [32] , [35] , hydroalkylation produces molecules that are richer in sp 3 -hybridized carbon centers and contain more stereogeometric information [36] , [37] , [38] , [39] , [40] , [41] , [42] , a feature that may improve biological activity [43] , [44] . In the 1990s, Mori disclosed intramolecular C(sp 3 )–C(sp 3 ) bond formation reactions between conjugated dienes and carbonyl groups with catalysis by a nickel hydride complex generated by treatment of Ni(cod) 2 with Et 3 SiH [45] . In the past 5 years, an array of elegant Ni-catalyzed hydroalkylation reactions between olefins and alkyl halides in the presence of a silane-based hydride source, including both enantiospecific and enantioconvergent versions, have been established (Fig. 1a ) [36] , [37] , [38] , [39] , [40] , [41] , [42] . In 2020, Koh’s group developed an aminoquinaldine-directed hydroalkylation reaction, in which one alkyl halide molecule provides an alkyl motif and another delivers a hydride via β-H elimination [46] . In addition to alkyl halides, imines or aldehyde can also be used as coupling partners for hydroalkylation reactions of tetrafluoroethylene with silanes [47] , [48] . Fig. 1: Nickel-catalyzed hydroalkylation of olefins. a Hydroalkylation of olefins with an additional hydride source. b An N-sulfonyl amine serves both as a hydride source and a coupling partner in the hydroalkylation of olefins. c Envisioned catalytic cycle and challenges. cat. catalyst, PCy 3 tricyclohexylphosphine, Ar aryl, Ts tosyl, Mts mesitylen-2-sulfonyl. Full size image Inspired by Ni-engaged oxidative cyclometallation ([Ni 0 ] to nickellacycle a in Fig. 1c ), which have been successfully applied in alkenylation of imines with unsaturated molecules such as alkynes and olefins [49] , [50] , [51] , [52] , [53] , [54] , [55] , [56] , we envisioned that if an amine could serve both as a hydride source and an imine precursor, formal olefin insertion into the α-C–H bond of the amine could be accomplished (Fig. 1c ). Although the Ni-catalyzed alkenylation reaction between alkynes and amines has been reported [57] , [58] , the above-described strategy poses a significant challenge in the form of competitive hydride elimination from one of the β-positions relative to the nickel atom ( b to c vs b to side product). For instance, the alkenylation reactions between olefins and imines established by Zhou’s group provided unsaturated products, allylic amines [54] . When tetrafluoroethene bearing no hydrogen atom was subjected together with silane, alkylation of imines took place [47] . Moreover, Ogoshi’s group recently used carbonyl insertion to interrupt the facile β-H elimination; displacement of the nickel from the nickellacycle intermediate provides saturated γ-lactams [59] , [60] . In this work, we report a Ni-catalyzed hydroalkylation of olefins with N-sulfonyl amines, which provides α-branched amines without the need for an exogenous hydride source, and obtains high enantioselectivity by using a P-chiral phosphine ligand (Fig. 1b ). Reaction optimization To evaluate the feasibility of our strategy, we selected N-tosyl benzylamine ( 1a ) and styrene ( 2a ) as coupling partners. We conducted the hydroalkylation by using a Ni(0) species Ni(cod) 2 and a phosphine ligand PCy 3 . After trying a number of weak inorganic bases (Fig. 2a ), including NaOAc and K 3 PO 4 , which are crucial in our previous studies [57] , we only detect a trace amount of the desired hydroalkylation product 3a together with a side-product allylic amine 3a’ by 1 H NMR spectroscopy. However, we found strong bases could dramatically promote the designed reaction profile, as well as suppress the competitive pathway that leads to 3a’ . For instance, KO t Bu provided 3a in an almost quantitative yield (98% NMR yield) with a 10 mol% Ni catalyst. Phenyl boronic acid is not necessary, but it influenced the efficiency of this catalysis that a lower yield (40%) was obtained in the absence of it. Moreover, we evaluated other boron reagents and found that 2-phenyl-1,3,2-dioxaborinane and its analogue bearing no protons also gave high yields (Fig. 2b ). Next, we moved to evaluate ligands beside PCy 3 , including monodentate and bidentate phosphines, as well as other type pivotal ligands: the analogues of PCy 3 , such as PCyp 3 (Cyp, cyclopentyl group) and PCy 2 Ph, yielded product 3a in around 70% yields; the use of other ligands resulted in much lower or even undetectable yields (Fig. 2c ). Fig. 2: Reaction optimization. a Evaluation of base. b Evaluation of boron reagent. c Evaluation of ligand. d Standard reaction conditions. e Gram-scale reaction. Reaction conditions: 1a (0.2 mmol), 2a (0.4 mmol), Ni(cod) 2 (10 mol%), ligand (20 mol%), PhB(OH) 2 (25 mol%), base (25 mol%), toluene (0.3 mL), N 2 , 120 °C; yields were determined by 1 H NMR spectroscopy. a Without PhB(OH) 2 . b Ligand (10 mol%). B boron, Ac acetyl, Bu butyl, Me methyl, TMS trimethylsilyl, KHMDS potassium bis(trimethylsilyl)amide, Ph phenyl, Pr propyl. Full size image Although nickel is more earth-abundant and much less expensive than precious metals (Pd, Rh, Ir, etc. ), carrying out reactions with less catalysts is vital from both an atom-economy and an environmentally friendly standpoint. Therefore, we carried out experiments with lower catalyst loadings and found that the loading of the nickel/phosphine catalyst could be reduced to 2.5 mol% with no obvious decrease in yield (Fig. 2d ). In addition, a gram-scale reaction with a nickel loading of only 1 mol% afforded 3a with no need for column chromatography (Fig. 2e ), and the protecting group (Ts) could be easily displaced by a Boc group (see Supplementary Methods 2.4 for details). Substrate scope With the optimized reaction conditions in hand, we investigated the generality of this method. First, we examined the scope of the reaction with respect to the N-tosyl amine (Fig. 3 ). A wide range of benzylic amines bearing an ortho ( 3b – d ), meta ( 3e – h ), or para ( 3i – r ) substituent on the aromatic ring underwent the coupling reaction with styrene ( 2a ), delivering the desired α-branched amines in 42–99% yields. Substrates with disubstituted phenyl rings ( 3s – t and 3v ) or a naphthyl ring ( 3 u ) were also well tolerated. Heterocycles containing an oxygen, sulfur, or nitrogen atom are prevalent in pharmaceuticals, but metal-catalyzed reactions involving such compounds are challenging because of coordination between the heteroatom and the metal. Indeed, we found that heteroatom-containing substrates gave low yields ( 3w – y ) under the standard conditions. When a higher loading of the catalyst (5 mol%) and an additive, pivaldehyde, were used, the reactions afforded the desired products in moderate yields. Fig. 3: Substrate scope of N-tosyl amines. Reaction conditions: N-sulfonyl amine 1 (0.2 mmol), 2a (0.4 mmol), Ni(cod) 2 (2.5 mol%), PCy 3 (5 mol%), PhB(OH) 2 (25 mol%), KO t Bu (25 mol%), toluene (0.3 mL), N 2 , 120 °C; isolated yields were reported. a Ni(cod) 2 (5 mol%), PCy 3 (10 mol%). b PhB(OH) 2 (100 mol%), KO t Bu (50 mol%). c Pivaldehyde (2.0 equiv.) was added. d Ni(cod) 2 (5 mol%), PCy 3 (10 mol%), PhB(OH) 2 (100 mol%), KO t Bu (100 mol%). Bz, benzoyl, Et ethyl, Boc tert -butyloxycarbonyl. Full size image In addition to benzylic amines, various primary aliphatic amines were also acceptable substrates under modified conditions. Substrates with linear ( 3z – af ), γ-branched ( 3ag – ai ), β-branched ( 3aj ), and cyclic ( 3ak – an ) alkyl groups at the α-position of the nitrogen were tolerated, affording the corresponding unsymmetrical α-branched amines in moderate to good yields. The scope of olefins was then examined with N-tosyl amine 1a (Fig. 4 ). Both electron-donating and -withdrawing groups on the phenyl rings of olefins were well tolerated; desired products 3ao – ba were obtained in moderate to excellent yields. Moreover, a diverse array of functionalities such as fluorine, trifluoromethyl, methoxy, ester, morpholino, and ketone were tolerated. Multisubstituted aryl olefins, including a molecule derived from estrone, were suitable substrates, affording 3ay – ba in good yields. Olefins containing a heterocycle, such as indole, benzofuran, and quinoline, as well as ferrocene were also compatible with the reaction conditions. In addition, hydroalkylation of aliphatic olefins with 1a in the presence of pivaldehyde provided mixtures of linear and branched products in 41–92% yields. Fig. 4: Substrate scope of olefins. Reaction conditions: 1a (0.2 mmol), olefin 2 (0.4 mmol), Ni(cod) 2 (2.5 mol%), PCy 3 (5 mol%), PhB(OH) 2 (25 mol%), KO t Bu (25 mol%), toluene (0.3 mL), N 2 , 120 °C; isolated yields were reported. a Ni(cod) 2 (5 mol%), PCy 3 (10 mol%). b PhB(OH) 2 (100 mol%), KO t Bu (50 mol%). c Pivaldehyde (2.0 equiv.) was added. d The ratio of linear product to branched product (l/b) was determined by 1 H NMR spectroscopy. Hex hexyl, Bn benzyl. Full size image We next investigated whether this protocol could be applied to access enantioenriched α-branched N-tosyl amines, which are valuable and privileged motif found in nature products, pharmaceuticals, and functional molecules. 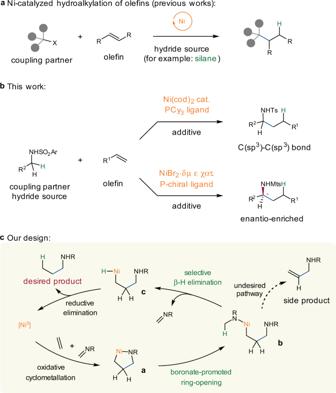Fig. 1: Nickel-catalyzed hydroalkylation of olefins. aHydroalkylation of olefins with an additional hydride source.bAn N-sulfonyl amine serves both as a hydride source and a coupling partner in the hydroalkylation of olefins.cEnvisioned catalytic cycle and challenges. cat. catalyst, PCy3tricyclohexylphosphine, Ar aryl, Ts tosyl, Mts mesitylen-2-sulfonyl. We immediately encountered a significant challenge in that a chiral ligand such as P-chiral phosphine ( R )-BI-DIME [61] together with Ni(cod) 2 , provided the desired product with a poor enantioselectivity (57.2:42.8 er) (see Supplementary Table 11 ). We suspected that the 1,5-cyclooctadiene (cod) liberated from Ni(cod) 2 may rebind to the metal center during the catalysis, leading to a disturbance in enantioselectivity control. To diminish such influence, we evaluated other Ni sources, and found that a Ni(II) precatalyst NiBr 2 ·dme, which could be reduced to Ni(0) in situ, dramatically improved the enantioselectivity (79.6:20.4 er). Instead of the tosyl group, using a bulkier mesitylen-2-sulfonyl group (Mts) as the protecting group for nitrogen resulted in a slightly better result (83.6:17.4 er). Further optimization of the conditions, including solvent and reaction temperature allowed us to obtain 5a in 55% isolated yield with 92.0:8.0 er (for more details, see Supplementary Table 11 ). Then, we move to investigate the substrate scope of the enantioselective protocol by performing reactions of aliphatic N-Mts amines with olefins (Fig. 5 ). First, various styrene analogues were compatible under the optimized conditions, providing desired products in moderate yields with good enantioselectivities ( 5a – n ). Second, the scope of amines is also broad that both acyclic ( 5o – aa ) and cyclic ( 5ab – af ) aliphatic amines were suitable. Notably, active functional groups, including ester ( 5s ), amide ( 5t ), imide ( 5u ), carbamate ( 5ae ), and cyclopropyl ( 5w ) were well tolerated. The absolute configuration of ( S )- 5n was determined by X-ray crystallography (see Supplementary Note 2 ). Fig. 5: Substrate scope of enantioselective hydroalkylation. Reaction conditions: 4 (0.1 mmol), olefin 2 (0.2 mmol), NiBr 2 ·dme (10 mol%), ( R )-BI-DIME (20 mol%), PhB(OH) 2 (120 mol%), KO t Bu (120 mol%), anisole (0.2 mL), N 2 , 60 °C; isolated yields were reported. a Reaction was conducted at 50 o C. b Reaction was conducted at 80 o C. c ( R )-BI-DIME (12 mol%) was used. Nap naphthyl, Oct octyl. Full size image Mechanistic studies To gain insights into the reaction mechanism, we performed mechanistic studies. First, we replaced amine 1a with N-tosyl imine 6a and found that the reaction yielded only a trace of desired product 3a (Fig. 6a ). Moreover, adding para -methoxybenzylamine ( 1 l ) to the above reaction mixture dramatically increased the yield of 3a . These experiments suggested that the N-tosyl amine served not only as the precursor of the imine but also as the hydride source to terminate the catalytic cycle. Second, deuterium-labeling experiments were conducted (Fig. 6b ). When the α-deuterated substrate 1u-d 2 was used, 45.5% average deuterium incorporation at the γ-position relative to the nitrogen of the product was detected, and the recovered substrate showed no loss of deuterium. This observation is consistent with our assumption that the hydrogen in the product was derived mainly from the N-tosyl amine. Third, control experiments were carried out to investigate the role played by pivaldehyde in the reactions of aliphatic olefins (Fig. 6c ). In the absence of the aldehyde, only a very low yield was obtained (<8%). In contrast, when an α,α,α-trisubstituted aldehyde α-naphthalenyl isobutyraldehyde 7 (Compared to pivaldehyde, α-naphthalenyl isobutyraldehyde and its corresponding alcohol are easier to observe by 1 H NMR spectroscopy) was used, 3bg was obtained in 57% yield, along with an alcohol derived from the aldehyde. Moreover, a catalytic amount of N-tosyl imine (10 mol%) also promoted the reaction, which indicates that the aldehyde additive may accept hydride from the Ni–H species generated in the initial step (N-tosyl amine dehydration), prior to catalysis. Fig. 6: Mechanistic studies. a Hydroalkylation of styrene with N-tosyl imine. b Deuterium labeling experiment. c Effects of an aldehyde in the hydroalkylation of 1-octene. Full size image In addition, we investigated effects of the base and boron reagent. First, a strong base such as KO t Bu, LiO t Bu, and KOMe was found to be indispensable; while, beside PhB(OH) 2 , a borate such as 2-phenyl-1,3,2-dioxaborinane also dramatically promoted the reaction (Fig. 2 ). Second, we used 11 B NMR to evaluate interactions between PhB(OH) 2 and reactants, including N-tosyl amine, styrene, and KO t Bu (Fig. 7 ). After heating the reaction mixture for a while (in the absence of Ni/P-catalyst), a new peak appeared in the upfield, implying the formation of a boronate complex. Notably, this peak still appeared either in the absence of an olefin or when PhB(OH) 2 was treated with potassium sulfonamide ( 8 ) directly. Furthermore, a boronate complex ( 9 ) bearing a B–N bond was isolated and characterized by NMR spectroscopy as well as elementary analysis ([C 20 H 21 BKNO 4 S], calcd. for B: 2.57%; found: 2.73%.). Beside KO t Bu, we subjected LiO t Bu into the above experiments, and also observed the formation of lithium boronate by 11 B NMR spectroscopy (see Supplementary Methods 2.6 for details). 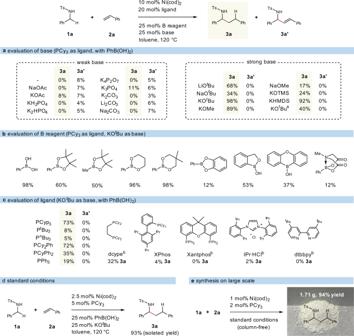Fig. 2: Reaction optimization. aEvaluation of base.bEvaluation of boron reagent.cEvaluation of ligand.dStandard reaction conditions.eGram-scale reaction. Reaction conditions:1a(0.2 mmol),2a(0.4 mmol), Ni(cod)2(10 mol%), ligand (20 mol%), PhB(OH)2(25 mol%), base (25 mol%), toluene (0.3 mL), N2, 120 °C; yields were determined by1H NMR spectroscopy.aWithout PhB(OH)2.bLigand (10 mol%). B boron, Ac acetyl, Bu butyl, Me methyl, TMS trimethylsilyl, KHMDS potassium bis(trimethylsilyl)amide, Ph phenyl, Pr propyl. Inspired by the previous observations that compounds bearing active protons (e.g. TsNH 2 , phenol) could promote opening of the five-membered nickellacycle intermediate via protonation [50] , [54] , [62] , [63] , [64] , as well as studies of transmetallation on boronates [65] , [66] , [67] , [68] , [69] , we proposed that a boronate facilitates exchange of the sulfonamidyl group on the nickel, leading to rapid opening of the nickellacycle ( a to b in Fig. 1c ). Fig. 7: 11 B NMR (toluene- d 8 ) studies. 11 B NMR spectroscopy was used to evaluate interactions between PhB(OH) 2 and reactants, including N-tosyl amine, styrene, and KO t Bu. Full size image On the basis of the aforementioned experiments and previous studies [49] , [50] , [51] , [54] , [56] , [57] , we proposed the mechanism outlined in Fig. 8 . The process is initiated by dehydrogenation of a N-sulfonyl amine, liberating a catalytic amount of the corresponding imine together with a Ni-H species. Subsequently, styrene or the additive pivaldehyde accepts hydride to regenerate the active Ni(0) catalyst. In the catalytic cycle, oxidative cyclometallation produces a nickellacycle intermediate Int 1 , which is converted into the nickel intermediate Int 2 through a boronate-promoted exchange of sulfonamidyl group. Finally, the desired product is derived from Int 2 through a β-H elimination/reductive elimination process, completing the catalytic cycle. Fig. 8: Proposed catalytic cycle. Possible reaction mechanism of the Ni-catalyzed hydroalkylation of olefins with N-sulfonyl amines. Full size image In summary, we have developed a method for nickel-catalyzed hydroalkylation reactions between terminal olefins and linear N-sulfonyl amines to afford a variety of branched products. The method is atom economical because an exogenous hydride source is not required. Mechanistic studies suggested that a sulfonamidyl boronate complex formed in situ facilitates the transformation by promoting the opening of the nickellacycle. Further work aimed at extending this protocol to related transformations is currently underway in our laboratory. General procedure for hydroalkylation of olefins with N-sulfonyl amines In a N 2 -filled glovebox, a 4 mL oven-dried vial was charged with N-sulfonyl amine 1 (0.2 mmol, 1.0 equiv. ), olefin 2 (0.4 mmol, 2.0 equiv. ), Ni(cod) 2 (0.005 mmol, 1.4 mg, 2.5 mol%), PCy 3 (0.01 mmol, 2.8 mg, 5 mol%), PhB(OH) 2 (0.05 mmol, 6.1 mg, 25 mol%) and KO t Bu (0.05 mmol, 5.6 mg, 25 mol%). Toluene (0.3 mL) was added. The vial was equipped with a magnetic stir bar, sealed, and the reaction mixture was stirred at 120 °C for 20 h. The reaction mixture was cooled to room temperature and concentrated under reduced pressure. Purification by column chromatography afforded the desired product. General procedure for enantioselective hydroalkylation of olefins with N-sulfonyl amines In a N 2 -filled glovebox, a 4 mL oven-dried vial was charged with N-sulfonyl amine 4 (0.1 mmol, 1.0 equiv. ), olefin 2 (0.2 mmol, 2.0 equiv. ), NiBr 2 ·dme (0.01 mmol, 3.1 mg, 10 mol%), ( R )-BI-DIME (0.02 mmol, 6.6 mg, 20 mol%), PhB(OH) 2 (0.12 mmol, 14.6 mg, 120 mol%) and KO t Bu (0.12 mmol, 13.4 mg, 120 mol%). Anisole (0.2 mL) was added. 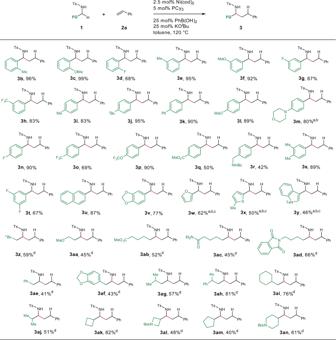Fig. 3: Substrate scope of N-tosyl amines. Reaction conditions: N-sulfonyl amine1(0.2 mmol),2a(0.4 mmol), Ni(cod)2(2.5 mol%), PCy3(5 mol%), PhB(OH)2(25 mol%), KOtBu (25 mol%), toluene (0.3 mL), N2, 120 °C; isolated yields were reported.aNi(cod)2(5 mol%), PCy3(10 mol%).bPhB(OH)2(100 mol%), KOtBu (50 mol%).cPivaldehyde (2.0 equiv.) was added.dNi(cod)2(5 mol%), PCy3(10 mol%), PhB(OH)2(100 mol%), KOtBu (100 mol%). Bz, benzoyl, Et ethyl, Boctert-butyloxycarbonyl. The vial was equipped with a magnetic stir bar, sealed, and the reaction mixture was stirred at 60 °C for 72 h. The reaction mixture was cooled to room temperature and concentrated under reduced pressure. 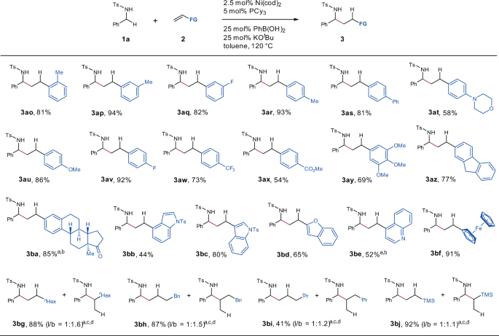Fig. 4: Substrate scope of olefins. Reaction conditions:1a(0.2 mmol), olefin2(0.4 mmol), Ni(cod)2(2.5 mol%), PCy3(5 mol%), PhB(OH)2(25 mol%), KOtBu (25 mol%), toluene (0.3 mL), N2, 120 °C; isolated yields were reported.aNi(cod)2(5 mol%), PCy3(10 mol%).bPhB(OH)2(100 mol%), KOtBu (50 mol%).cPivaldehyde (2.0 equiv.) was added.dThe ratio of linear product to branched product (l/b) was determined by1H NMR spectroscopy. Hex hexyl, Bn benzyl. 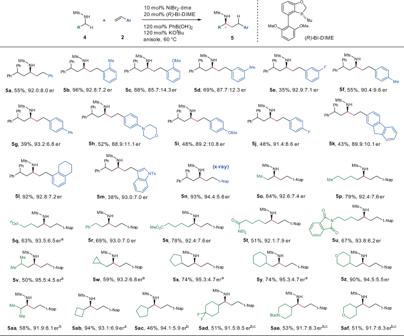Fig. 5: Substrate scope of enantioselective hydroalkylation. Reaction conditions:4(0.1 mmol), olefin2(0.2 mmol), NiBr2·dme (10 mol%), (R)-BI-DIME (20 mol%), PhB(OH)2(120 mol%), KOtBu (120 mol%), anisole (0.2 mL), N2, 60 °C; isolated yields were reported.aReaction was conducted at 50oC.bReaction was conducted at 80oC.c(R)-BI-DIME (12 mol%) was used. Nap naphthyl, Oct octyl. 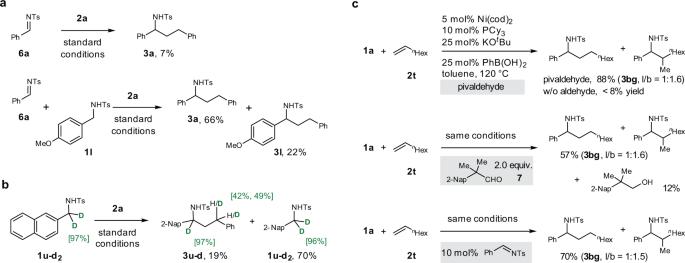Fig. 6: Mechanistic studies. aHydroalkylation of styrene with N-tosyl imine.bDeuterium labeling experiment.cEffects of an aldehyde in the hydroalkylation of 1-octene. 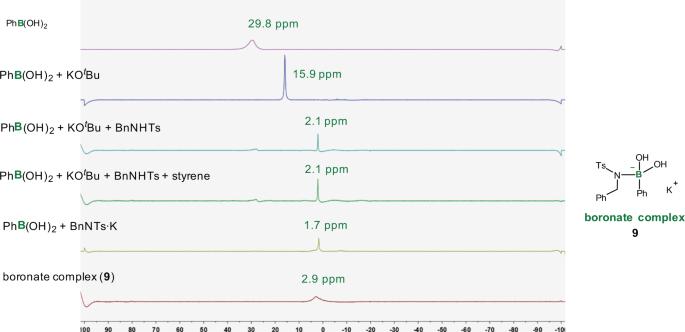Fig. 7:11B NMR (toluene-d8) studies. 11B NMR spectroscopy was used to evaluate interactions between PhB(OH)2and reactants, including N-tosyl amine, styrene, and KOtBu. 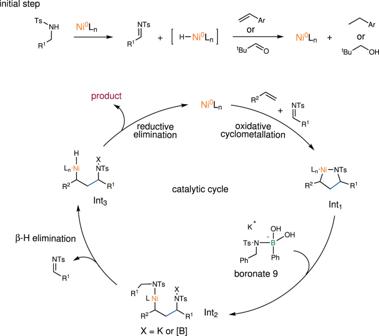Fig. 8: Proposed catalytic cycle. Possible reaction mechanism of the Ni-catalyzed hydroalkylation of olefins with N-sulfonyl amines. Purification by column chromatography afforded the desired product.